Topological defect formation and spontaneous symmetry breaking in ion Coulomb crystals Symmetry breaking phase transitions play an important role in nature. When a system traverses such a transition at a finite rate, its causally disconnected regions choose the new broken symmetry state independently. Where such local choices are incompatible, topological defects can form. The Kibble–Zurek mechanism predicts the defect densities to follow a power law that scales with the rate of the transition. Owing to its ubiquitous nature, this theory finds application in a wide field of systems ranging from cosmology to condensed matter. Here we present the successful creation of defects in ion Coulomb crystals by a controlled quench of the confining potential, and observe an enhanced power law scaling in accordance with numerical simulations and recent predictions. This simple system with well-defined critical exponents opens up ways to investigate the physics of non-equilibrium dynamics from the classical to the quantum regime. Phase transitions are ubiquitous in nature, from the freezing of water to the emergence of superfluidity, superconductivity and ferromagnetism, as well as symmetry breaking in cosmology [1] , [2] . In particular, the universality of second-order phase transitions makes their dynamics largely independent from their microscopic nature. This has led to a comprehensive effort to study them in a wide range of systems [1] , [2] , [3] , [4] , [5] , [6] , [7] , [8] , [9] , [10] . These studies test a theory of second-order phase transition dynamics, the Kibble–Zurek mechanism (KZM), that predicts the scaling of defect formation with quench rate. In previous experiments, this scaling was studied primarily in homogeneous systems, such as in fluxoid formation in superconducting loops [5] and ferroelectric domains in multiferroics [6] . A more complete overview on KZM experiments can be found in Supplementary Note 1 . The main difficulty with observing the KZM scaling is the weak fractional power law dependence of defect densities that requires varying the control parameter over a large range to obtain a high sensitivity to the scaling exponent. This means that one has to change the quench time over orders of magnitude to gain a reliable signal. A way to enhance the scaling of defect density on quench rate that relies on causality (central to KZM) was suggested [3] for investigation of systems in harmonic traps. Here, symmetry breaking begins in the centre of the trap, and the transition front propagates with a speed set by the quench rate and the local gradient of the potential. Where the front is faster than the relevant speed of sound, different parts of the system cannot communicate and they break symmetry independently as in the case of a homogeneous transition [11] , [12] . However, further from the trap centre, the phase front slows, and as it becomes slower than the speed of sound defect production ceases (as the outlying parts of the system inherit broken symmetry from their neighbours). Thus, in harmonic traps the quench rate controls both the density of defects in the homogeneous region and the size of the fraction of the trap in which they can be produced. This leads to steeper scalings [3] , [4] , [13] . Here, we use chains of ions confined in harmonic traps that present a promising platform for quantum simulation and information processing [14] , [15] , [16] , [17] , [18] as a well-controlled system to study the dynamics of symmetry breaking and the formation of topological defects. This system offers excellent experimental control over the quench rate of the trapping potential and offers the possibility of studying defect formation in a setting in which the sensitivity is improved due to the enhanced scaling that occurs in inhomogeneous systems [3] , [4] . In contrast to previous experiments, no assumptions regarding the values of the critical exponents are necessary, as they can be derived using the Ginzburg–Landau model [4] . In this study, we present the creation of stable topological defects in ion Coulomb crystals and measure the scaling of defect creation with respect to the controlled quench parameter as compared to the predictions of the KZM theory. Scaling of defect creation in a harmonic ion trap Our experiment tests a theory—the KZM [1] , [2] —that employs equilibrium scaling behaviour to predict their non-equilibrium consequences. Critical slowing down, that is, the divergence of the relaxation time of the system, implies that every second-order phase transition traversed at a finite rate will inevitably depart from equilibrium near the critical point, where a discrete symmetry is chosen. In a trapped ion chain, as the triaxial confining potential is weakened in the transverse direction, the chain buckles and the ions form a ‘zigzag’ (see Fig. 1 ). This breaking of the (axial) symmetry is a second-order phase transition described by the Ginzburg–Landau theory [19] . It can lead to the formation of topological defects (for example, places where a ‘zig’ is followed by another ‘zig’ rather than a ‘zag’), as highlighted in Fig. 1 by red circles. Depending on the speed at which the transverse potential is quenched, the system chooses a final configuration of either a pure ‘zigzag’ or kinks dividing the two different orientations with a certain probability. The appearance of such kinks, that show soliton-like behaviour [20] , is a result of the incompatible local choices of symmetry breaking. 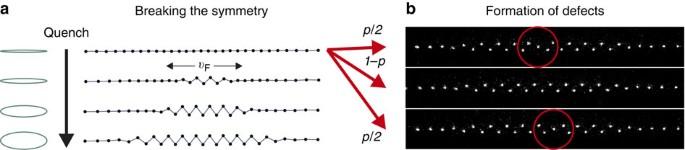Figure 1: Phase transition in an inhomogeneous system leading to kink formation. (a) An ion chain buckles in the centre and the ‘zigzag’ region spreads at a finite velocity υFduring a quench of the transverse confinement (illustrated by the green ellipses). (b) Examples of the configuration after a quench: normal ‘zigzag’ (centre) and kink and anti-kink (top and bottom). The system chooses the final configuration with a certain probability, depending on the speed at which the phase transition is crossed. Figure 1: Phase transition in an inhomogeneous system leading to kink formation. ( a ) An ion chain buckles in the centre and the ‘zigzag’ region spreads at a finite velocity υ F during a quench of the transverse confinement (illustrated by the green ellipses). ( b ) Examples of the configuration after a quench: normal ‘zigzag’ (centre) and kink and anti-kink (top and bottom). The system chooses the final configuration with a certain probability, depending on the speed at which the phase transition is crossed. Full size image In the thermodynamic limit, near second-order phase transitions, the relaxation time τ and the healing length ξ (which set the time and the length scales on which the order parameter returns to its equilibrium value) diverge as τ = τ 0 /|ε| νz and ξ = ξ 0 |ε| v as the dimensionless distance ε to the critical point approaches zero. Here, τ 0 and ξ 0 depend on the microphysics, while the critical exponents v and z define the universality class of the transition. The distance from the critical value is given by the dimensionless parameter , where λ c is the critical value of the control parameter λ at which the phase transition occurs. The change of ε with time takes the system from the symmetric (ε<0) to the symmetry-broken (ε>0) phase. In what follows, we take ε= t / τ Q , where τ Q is the timescale on which the phase transition is crossed. The ratio of ξ and τ yields the speed of sound at which the information about the choice of broken symmetry can propagate. The size of domains that can coordinate symmetry breaking is set at the instant when, because of critical slowing down, the state of the system ceases to follow changes imposed by the time-dependent control parameter ε. This happens when the relaxation time τ matches the timescale of the changes imposed on the system. This time, , determines the size of the domains , that is, the typical separation between topological defects. In del Campo et al . [4] , Coulomb crystals trapped in a harmonic axially confining potential were proposed to measure the scaling of defect formation to test KZM. In such crystals, the charge density along the ion chain is larger in the centre and reduces towards the edges. Within the local density approximation, this inhomogeneity is inherited by the critical control parameter λ c . In our case, this control parameter is the transverse secular frequency ν t describing the radial confinement. The spatial dependence of its critical value is given by . Here, ω ( x ) is the characteristic frequency of the axial Coulomb coupling along the trap axis x . It is given in terms of the mass m and charge Q of the ion, and the axial inter-ion spacing a ( x ), which reaches its minimum value at the centre of the ion chain, that is, at x =0. Laser cooling provides a dissipative force acting on the ions described by the friction parameter η (for a definition of η and its experimental parameters, see Methods ). In the underdamped regime accessible in our experiment, the characteristic response time is fixed by the inverse of ω (0) and the sound velocity becomes independent of η (and x ). As a result, the system exhibits mean-field critical exponents v =1/2 and z =1 (see del Campo et al . [4] ). We consider a quench of the transverse secular frequency of amplitude δ in a timescale τ Q , that is, . During the quench, the phase transition is first crossed at the centre of the chain. The velocity of the front υ F with which the critical point propagates depends on the quench rate and varies along the chain. The dynamics of an inhomogeneous phase transition is governed by the interplay of υ F and the sound velocity υ . For extremely fast quenches, the inequality υ F > υ holds everywhere in the system, and the paradigmatic KZM for homogeneous systems is recovered. The sharpness of this inequality was studied in detail (see Supplementary Note 2 ). In this regime the density of kinks d scales with the quench rate as , in agreement with the KZM. At lower quench rates, υ F > υ is only satisfied in a fraction of the system, which depends on the quench rate. This results in an effective system size , where defects can be produced with densities predicted by KZM [3] , [4] . Outside this spatial region, the critical front is slower than υ , and defects will not form [11] . As a result of this interplay between propagating phase front and finite speed of sound, the total number of kinks in the inhomogeneous KZM is substantially reduced and exhibits a more pronounced dependence on the quench rate, that is, , see Fig. 2 . 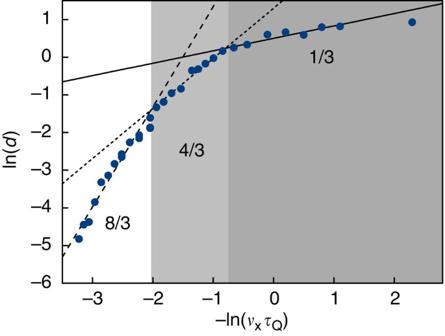Figure 2: Three regimes of kink creation. Numerical simulation of the created kink densitydin a 30-ion Coulomb crystal as a function of the quench timeτQusing experimental trap frequenciesνx/2π=24.6 kHz,νt/2π=500–140 kHz and a friction parameter ofη=1.5 × 10−20kg s−1. The simulations suggest three regimes governed by the sound and front velocities as indicated by the plotted lines with slopes of 1/3, 4/3 and 8/3, respectively. The quench rate is scaled in units of the axial secular frequencyνxω(0). Each data point represents more than 2,000 samples and has an error of <5% except for quenches with ln[1/(νxτQ)]<−2.5, where the error is 10–20% due to low kink creation rates. Figure 2: Three regimes of kink creation. Numerical simulation of the created kink density d in a 30-ion Coulomb crystal as a function of the quench time τ Q using experimental trap frequencies ν x /2π=24.6 kHz, ν t /2π=500–140 kHz and a friction parameter of η =1.5 × 10 −20 kg s −1 . The simulations suggest three regimes governed by the sound and front velocities as indicated by the plotted lines with slopes of 1/3, 4/3 and 8/3, respectively. The quench rate is scaled in units of the axial secular frequency ν x ω (0). Each data point represents more than 2,000 samples and has an error of <5% except for quenches with ln[1/( ν x τ Q )]<−2.5, where the error is 10–20% due to low kink creation rates. Full size image In finite-sized systems, τ and ξ , that diverge to infinity in an infinite system, ‘round off’ near the critical point. However, sufficiently far away from criticality the system will still behave like an infinite system [21] . This is the regime of relevance to the KZM, according to which the phase of the broken symmetry is chosen at the freeze-out time , away from the critical point. We have carried out numerical simulations with 30–100 ions to check how the defect scaling depends on the system size (the simulation for our experimental system with 30 ions is shown in Fig. 2 ). We consistently observe a linear KZM scaling indicating homogeneous and inhomogeneous regimes. For parameters such that a quench leads to only one or no defects, a steeper scaling is observed, see Fig. 2 . For this condition, a doubling of the Kibble–Zurek scaling has been reported previously in homogeneous systems in a series of works [5] , [22] , [23] . In the inhomogeneous case, when the kink density d becomes approximately equal to the probability to observe a single kink, this suggests a scaling of . Further details of the inhomogeneous regime can be found in Supplementary Note 2 . Creation of topological defects in ion Coulomb crystals In ion Coulomb crystals, two types of metastable defect configurations that are robust against thermal fluctuations have been identified in numerical simulations, that is, odd and extended kink solitons [4] , [20] . Experimentally, spontaneous kink formation has been observed during the process of crystallization induced by laser cooling [24] , [25] . In our experiment, we laser cool about 30 172 Yb + ions into a linear crystal in a three-dimensional harmonic trap [26] and create kinks via a controlled quench of the radial potential, see Methods section. We induce a slight ellipticity in the radial trapping frequencies and to confine the ions to a plane, and sweep both frequencies linearly over the critical value. In the final zigzag configuration, 1.3. The phase transition is governed by the lower transverse frequency . The structure of the Coulomb crystals is then detected and analyzed by imaging the fluorescence of the ions onto a camera. 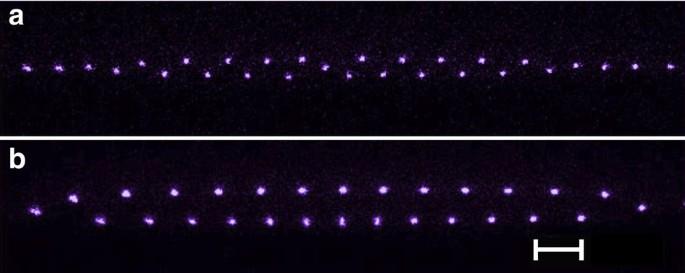Figure 3: Pictures of experimentally realized kinks in ion crystals. (a) Odd kink, created in shallow quenches (νt/2π=500–204 kHz). (b) Extended kink, observed for deep quenches of the radial frequency fromνt/2π=500–140 kHz. Exposure times are 50 and 200 ms, respectively. The Coulomb crystals consist of 29 (a) and 32 (b) ions and the phase transition sets in atνt,c/2π≈275 kHz. For the statistics measurements, we use the extended kink configuration to preserve and stabilize the created localized odd kinks. The scale bar indicates a length of 20 μm. Figure 3 shows the experimentally obtained stable configurations of both types of kinks. Figure 3: Pictures of experimentally realized kinks in ion crystals. ( a ) Odd kink, created in shallow quenches ( ν t /2π=500–204 kHz). ( b ) Extended kink, observed for deep quenches of the radial frequency from ν t /2π=500–140 kHz. Exposure times are 50 and 200 ms, respectively. The Coulomb crystals consist of 29 ( a ) and 32 ( b ) ions and the phase transition sets in at ν t,c /2π≈275 kHz. For the statistics measurements, we use the extended kink configuration to preserve and stabilize the created localized odd kinks. The scale bar indicates a length of 20 μm. Full size image For quench times, t =2 τ Q in the order of the oscillation period T =1/ ν x of the axial secular motion of the ions, kink formation in the two-dimensional ‘zigzag’ structure is observed as a break in the periodic order of the position of the ions. Depending on the final radial inter-ion spacing, odd or extended kink configurations are stable. The statistics described in this work is based on measurements of extended kinks, as in this configuration, the energy barrier for a defect, that is, the Peierls–Nabarro potential [27] , is larger and gives an inherently higher stability compared with odd kinks. As extended kinks are a result of initially created odd kinks during the radial quench and no more than one defect per quench is created in our experimental regime, both final configurations show the same statistics. This allows us to use extended kinks to test KZM scaling. In Supplementary Movies 1–3 , we show the experimental creation of odd and extended kinks, as well as a simulation of the time-resolved transformation of a odd kink into an extended kink. To obtain the statistics of kink formation, the radial quench cycle is repeated up to 4,400 times for each quench time and the density of defects d is defined as the average number of kinks per quench cycle. We measure the kink density as a function of the quench time τ Q at a fixed axial frequency ν x /2 π =24.6±0.5 kHz. The kink densities obtained in our experiment range from 0.01 to 0.24, that is, from one kink, for every 100 quenches, to another kink for every 4–5 quenches. The ultra-high vacuum with a pressure of 5 × 10 −9 Pa assures a low rate of spontaneous kink formation due to melting and recrystallization after background gas collisions. We experimentally determined the rate as one kink in 67 s of observation time in the ‘zigzag’ configuration. This allows the detection of kinks created in a controlled quench down to a minimum probability of 6 × 10 −4 , corresponding to ln( d )=−7.4. Collisions also limit the lifetime of our kinks that were experimentally determined to be 1.6 s (see Supplementary Fig. S1 ). Kink dynamics simulations and analysis of observed scaling In finite systems, losses can occur not only when pairs of kinks annihilate but also when kinks move out of the ‘zigzag’ region. The Peierls–Nabarro potential of the initially created odd kinks builds up during the quench from the centre and decreases to zero towards the outer linear parts of the crystal. The mobility of kinks is determined by the depth of this potential in comparison with their kinetic energy, which is gradually dissipated by the phononic coupling to the laser-cooled crystal at a rate quantified by the friction parameter η . Once a kink is able to change sites, it experiences an outward acceleration due to the inhomogeneity of the potential, enhancing the losses. We performed numerical simulations to investigate the dynamics that can lead to losses of kinks before they can be detected experimentally. As a result, we have identified two regimes: (1) for very slow quenches, losses occur due to the fact that defects escape into the linear region before the confining potential has built up sufficiently, and (2) for fast quenches, an enhanced amount of kinetic energy is introduced into the system that allows defects to leave the ‘zigzag’ region even after the quench has completed. To separate the effect of these losses from the density of kinks predicted by KZM, the time evolution of the number of defects for each quench cycle is determined in our simulations. We compared the absolute density of defects created during one cycle with the density of defects that remained after the ion motion has been damped out by the optical cooling forces (depending on the value of η , that is, at 350–500 μs after the radial quench). After this time, a constant number of defects is observed in the simulations, defining the density of stable kinks that are detectable in our experiment. 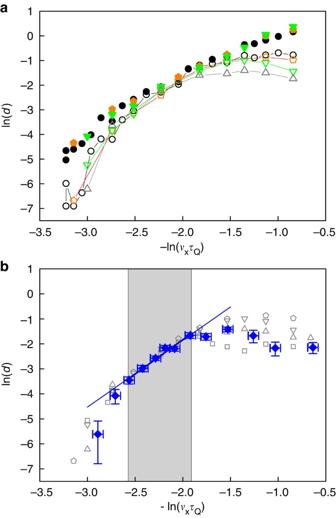Figure 4: Comparison of experimental data to simulations. (a) Numerical simulation of kink losses. Filled symbols show the number of kinks created during a radial quench. Open symbols are kinks remaining at the time of detection, where the lines are drawn to guide the eye. The symbols correspond toη=1.5 × 10−20kg s−1(circles), 6.0 × 10−21kg s−1(pentagons), 4.0 × 10−21kg s−1(inverted triangles) and 3.0 × 10−21kg s−1(triangles). The filled circles show the same data asFig. 2. (b) Experimentally measured kink density (filled symbols) compared with simulated density of kinks remaining at the time of detection forη=6.0 × 10−21kg s−1(pentagons), 4.0 × 10−21kg s−1(inverted triangles), 3.0 × 10−21kg s−1(triangles) and 2.5 × 10−21kg s−1(squares). The shaded region indicates the quench times for which kinks are stable and detectable in our experiment, and the blue line is the fit to the data points in this region. The vertical error bars include the s.e.m. of measurements repeated up to 4,400 times per data point over several months, as well as the statistical uncertainty assuming a binomial distribution. Horizontal error bars are because of the uncertainty in the axial-trapping frequency and a non-linear distortion of the applied ramp. Figure 4a shows the simulation results for the created and experimentally detectable kink densities for different values of η . There is a region with negligible losses from ≈−2 to ≈−2.5, where the experimental detection allows us to directly observe the density of created kinks. This is the region we use to compare the scaling of the measured kink density with the KZM predictions. The most important aspect regarding KZM tests, seen in Fig. 4a , is the independence of the density of created kinks (filled symbols) from the friction coefficient η . This proves that the phase transition happens in the underdamped regime, with well-defined dynamical critical exponent, z =1, see del Campo et al . [4] Figure 4: Comparison of experimental data to simulations. ( a ) Numerical simulation of kink losses. Filled symbols show the number of kinks created during a radial quench. Open symbols are kinks remaining at the time of detection, where the lines are drawn to guide the eye. The symbols correspond to η =1.5 × 10 −20 kg s −1 (circles), 6.0 × 10 −21 kg s −1 (pentagons), 4.0 × 10 −21 kg s −1 (inverted triangles) and 3.0 × 10 −21 kg s −1 (triangles). The filled circles show the same data as Fig. 2 . ( b ) Experimentally measured kink density (filled symbols) compared with simulated density of kinks remaining at the time of detection for η =6.0 × 10 −21 kg s −1 (pentagons), 4.0 × 10 −21 kg s −1 (inverted triangles), 3.0 × 10 −21 kg s −1 (triangles) and 2.5 × 10 −21 kg s −1 (squares). The shaded region indicates the quench times for which kinks are stable and detectable in our experiment, and the blue line is the fit to the data points in this region. The vertical error bars include the s.e.m. of measurements repeated up to 4,400 times per data point over several months, as well as the statistical uncertainty assuming a binomial distribution. Horizontal error bars are because of the uncertainty in the axial-trapping frequency and a non-linear distortion of the applied ramp. Full size image In Fig. 4b , the experimentally measured densities are shown, compared with simulated results for various values of η . A power law fit to the experimental data in the region from ln[1/( ν x τ Q )]=−1.9 to −2.6 yields a scaling of σ =2.7±0.3. This is in good agreement with the value of σ =2.63±0.13 obtained in a fit to the numerical data for the amount of kinks created (filled symbols in Fig. 4a ) from ln[1/( ν x τ Q )]=−2 to −3.2. The matching amount of losses at fast quenches is consistent with the assumed friction coefficient in the simulations. The data were taken over months with a repeatability indicated by the error bars. For quench times ln[1/( ν x τ Q )]<−1.7, the probability to produce more than one kink per ion chain becomes negligible. This corresponds to the regime in which the scaling coefficient is doubled to σ =8/3≈2.67, which is in agreement with the observed values in both experiment and simulations. We have demonstrated kink creation in the linear-to-‘zigzag’ structural phase transition in ion Coulomb crystals and studied its dependence on the quench rate of the trapping potential in a regime in which a maximum of one defect is created. In this regime, we have observed a doubling of the inhomogeneous scaling. The observed defect creation in our harmonic ion trap shows the influence of inhomogeneities in phase transitions, where the role of causality is enhanced and the formation of defects is suppressed by orders of magnitude compared with homogeneous systems. The experimentally accessible regime could be extended by enlarging the size of the crystal and by increasing the friction due to laser cooling. In this way, future experiments with Coulomb crystals may be able to measure the scaling in the other two regimes shown in Fig. 2 . Accessing the inhomogeneous KZM regime requires a larger system size in which it is easier to create more than one kink per chain. In order to avoid long-range interactions between defects, one could exploit the properties of the more localized odd kinks. Calculations of the Peierls-Nabarro potential of the different types of kinks will allow identification of optimum ion numbers, trap parameters to reduce losses and enable stable trapping of multiple kinks [28] , [29] . Experimental limitations in the system size can be overcome by using, for example, cryogenic ion traps that allow storage of large Coulomb crystals with long lifetimes [30] . The homogeneous KZM scaling could be tested with ions trapped in ring trap geometries [31] or linear ion traps with anharmonic axial confinement [32] . Our results open up ways to explore the various properties of discrete non-linear stable excitations, which have attracted considerable theoretical and experimental effort [33] . In such systems, the often counter-intuitive non-linear physics of solitons, breathers and their thermal fluctuations becomes accessible. Furthermore, to reach the onset of quantum effects in the phase transition, temperatures of a few tens of microkelvin, low-heating rates on the order of a hertz and possibly the use of a lighter ion species are required [34] , [35] . By implementing recently demonstrated advanced laser-cooling methods to prepare chains of ions [36] , [37] , [38] in the ground-state and ion traps with sub-hertz heating rates [39] , this work could be extended to study phase transitions in the quantum regime [40] . During the preparation of this manuscript, we became aware of similar results presented in another paper [41] . Atomic system and ion trap technology We laser-cool 172 Yb + ions on the 2 S 1/2 – 2 P 1/2 transition at a wavelength of 370 nm to temperatures of a few mK, slightly above the Doppler cooling limit [42] of T =0.5 mK for this transition. Two repump lasers at wavelengths 935 and 638 nm deplete the populations of higher lying metastable states that are coupled to the cooling cycle via radiative decay or collisions. A single coil on top of the vacuum chamber produces a quantization field of about B =0.2 mT at the ion position to optimize the repumping efficiency of the 935 nm laser. A detailed description of the experimental setup can be found in Pyka et al . [26] Laser cooling the ions via a single travelling wave leads to a friction coefficient of the optical cooling force given by at Δ=−Γ/2 (see Metcalf and van der Straten [42] ), where s is the saturation of the cooling transition, k is the wave vector of the cooling laser and Δ is the detuning of the laser with respect to the resonance of the transition with line width Γ. The transverse beam profile is focused down to horizontal and vertical waist sizes ω x =8.8 mm and ω y =80 μm. For a laser power of 630 μW, this results in an estimated experimental friction coefficient of η exp =4 × 10 −21 kg s −1 along a single axis. The simulations that have been carried out apply a friction parameter η sim to each axis and show the most agreement with the experiment for η sim =(2.5…3.0) × 10 −21 kg s −1 . The ion trap is a three-dimensional segmented linear radio frequency (rf) Paul trap, which was designed for high-precision spectroscopy on linear ion crystals. It offers full control to compensate stray fields in three dimensions and, in particular, has low axial micromotion over a large range of several hundreds of micrometres [26] . The ions are trapped in a loading segment via photoionization and then shuttled to a spectroscopy segment that is protected from the atomic beam. Avoiding contamination of the electrodes makes it possible to perform measurements with highly reproducible experimental parameters. The axial and radial secular frequencies in this segment were measured repeatedly, and a maximum deviation of σ ax =0.5 kHz and σ rad =1 kHz over several weeks was observed. For a linear crystal of about 30 ions with length l ~300 μm, the maximum axial rf field component along the crystal is as low as 500 V m −1 , whereas the radial field does not exceed 200 V m −1 corresponding to a total micromotion amplitude of only x mm =12 nm. The ion crystal is imaged with a self-built lens system optimized for minimum aberrations onto an electron multiplying CCD camera with a magnification of M =28 and an experimentally estimated resolution of about 1.5 μm over the full ion chain length of 300 μm. At the given axial trap frequency, about 30 ions can be imaged in the zigzag configuration. Radial quench cycle The rf voltage driving the radial confinement is amplitude modulated by a control signal using an rf mixer. Its actual amplitude on the ion trap electrodes is monitored by a short antenna inside the helical resonator ( U mon ), the impedance of which matches the amplified rf voltage U rf to the trap capacitance [26] . By observing parametric heating of the ions, we can measure the radial as well as axial secular frequencies directly as a function of the trap voltages with a relative precision of 10 −3 . To drive quenches of the radial confinement, a linear function, shown schematically in Supplementary Fig. S2 , is applied as a control signal to the rf mixer. Owing to the characteristics of the mixer, the measured slope of the ramp deviates from the ideal slope, and therefore is fitted to the monitored signal U mon (see Supplementary Fig. S3 ) to obtain the effective quench time used in the analysis as shown in Fig. 4b . The characteristic time constant of the resonant circuit of 7 μs limits the fastest possible quench time, but its effect on the ramps used in this work is negligible. The ramp has also been tested for linearity in trap frequency by verifying that a linear fit to the ramp near the point of the linear zigzag transition deviates by <2% from an ideal linear function between the frequencies measured at the extreme values of the ramp, see Supplementary Fig. S4 . Data analysis and statistics For each quench time, up to 4,400 pictures are taken in several series of measurements over 3 months. Accounting for this, the kink density for each quench time is calculated as the mean of the densities from the individual series for that time weighted by the number of pictures per series. The first and the biggest contribution to the error bars is the scatter of the individual series at a given quench time, calculated as sample s.d. The second and the independent contribution accounts for statistical uncertainty of the data, assuming a binomial distribution. Numerical simulations For Doppler cooled ions, the energy distribution of the ion chain obeys the Fokker–Planck distribution [43] . Hence, the dynamics of the j th ion can be described by the Langevin equation: where is the ponderomotive trapping potential, is the Coulomb potential energy, η is the friction coefficient due to laser cooling and ε j ( t ) is the stochastic force. The amplitude of the stochastic force, ε j ( t ), is related to the temperature T and the friction coefficient η by the fluctuation-dissipation relation ‹ ε α j ( t ) ε βk ( t ′)›=2 η k B Tδ αβ δ ij δ ( t−t ′ ), with α , β = x , y , z . Collisions with background particles are not included in this model. To simulate the quench from a linear-to-zigzag chain, the radial trapping frequencies, and , decrease linearly with time at rates corresponding to the experimentally measured values. The stochastic differential equation (1) was numerically integrated between 1,500 and 3,000 times per quench time τ Q in order to achieve a low statistical uncertainty. How to cite this article: Pyka, K. et al . Topological defect formation and spontaneous symmetry breaking in ion Coulomb crystals. Nat. Commun. 4:2291 doi: 10.1038/ncomms3291 (2013).